A general mechanism for competitor-induced dissociation of molecular complexes The kinetic stability of non-covalent macromolecular complexes controls many biological phenomena. Here we find that physical models of complex dissociation predict that competitor molecules will, in general, accelerate the breakdown of isolated bimolecular complexes by occluding rapid rebinding of the two binding partners. This prediction is largely independent of molecular details. We confirm the prediction with single-molecule fluorescence experiments on a well-characterized DNA strand dissociation reaction. Contrary to common assumptions, competitor-induced acceleration of dissociation can occur in biologically relevant competitor concentration ranges and does not necessarily imply ternary association of competitor with the bimolecular complex. Thus, occlusion of complex rebinding may play a significant role in a variety of biomolecular processes. The results also show that single-molecule colocalization experiments can accurately measure dissociation rates despite their limited spatiotemporal resolution. Non-covalent association of molecules in solution with proteins and nucleic acids underlies the function of biological systems. Quantitative understanding of the mechanisms by which these systems function requires measuring and interpreting the formation and dissociation kinetics of these non-covalent complexes. In the chemical and biochemical literature, non-covalent association and dissociation reactions are frequently approximated as systems that exist in two states, a bound state where the complex is formed and a free state in which the two binding partners are separate and can diffuse independently [1] . In these models, the free state is assumed to correspond to a well-mixed solution in which the concentration of the partners is uniform throughout. However, it is well established that the well-mixed solution assumption is not correct in all cases. For example, there are extensive precedents in research on ligand dissociation from cell surfaces with a high density of receptors [2] , [3] , [4] , [5] , [6] . In such systems, immediately after a ligand dissociates from a receptor it is still in the neighbourhood of the cell surface that may have many unoccupied receptors nearby. This ligand is thus more likely to rapidly rebind to a receptor on the cell surface than is a ligand in the bulk solution. Such rapid rebinding events make the dissociation of the ligand from the cell slower than the dissociation from a single receptor. In these systems, the apparent dissociation rate constant of ligand is increased by the presence of a competitor molecule that occupies adjacent receptors and thereby prevents rebinding of the ligand. Similar results have been obtained on other systems that involve closely spaced arrays of binding sites, for example, sequence nonspecific binding of proteins to DNA [7] . In contrast to systems with multiple closely spaced binding sites, the dissociation rate of an isolated bimolecular complex is in general assumed to be independent of competitor concentration. This expectation is frequently met by experimental results. In fact, when competitor dependence is observed [8] , [9] , [10] , [11] , the phenomenon is attributed to the transient formation of a ternary complex between the two binding partners and the competitor [12] , [13] , even in systems where independent evidence for the ternary complex is lacking. In this paper we consider an alternative explanation that even the dissociation of isolated bimolecular complexes is affected by rapid rebinding. In particular, we ask whether competitor acceleration of bimolecular complex dissociation is a general phenomenon that is expected even for molecules that do not form a ternary complex with competitor. To approach this problem, we apply previously developed models of bimolecular complex dissociation that are more physically realistic than the well-mixed solution model [14] , [15] , [16] , [17] . The more realistic models take into account diffusional separation of binding partners and the possibility they may rebind before complete mixing. We use these approaches to examine the effect of competitor on complex dissociation kinetics. These analyses predict that the dissociation rate constant in general depends on competitor concentration, even in situations when a ternary complex between the two binding partners and competitor does not form. In particular, the predicted effect does not depend on the molecular details of the interactions between the two binding partners. This general prediction is confirmed in experiments on a specific model reaction, the dissociation of a duplex DNA, using single-molecule fluorescence microscopy methods that are directly capable of observing dissociation in the absence as well as in the presence of competitor. Modeling competitor effect on molecular complex dissociation Physical understanding of the binding and dissociation processes is based on the concept of a free-energy landscape, in which the system moves along a multi-dimensional free-energy surface [18] , [19] . A freely diffusing molecule that is far away from its binding partner approaches the partner by diffusion. At small separations between the partners, the free energy of the system typically increases due to a variety of factors including adoption of restricted orientations of the partners, selection of rare molecular conformations and the possible need to desolvate binding surfaces. This free-energy increase is represented as an activation barrier for binding (Δ G a ‡ ). 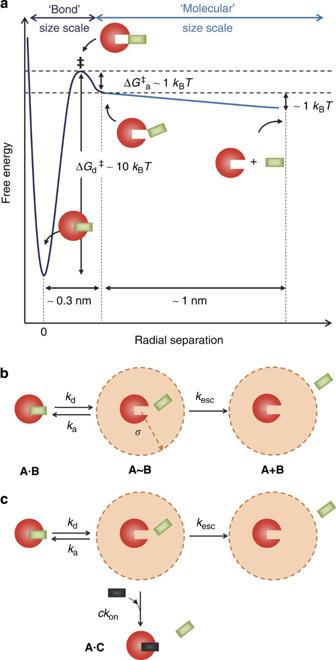Figure 1: Rapid rebinding of a bimolecular complex before full dissociation. (a) Schematic energy diagram for two binding partner molecules arbitrarily designatedA(red) andB(green) dissociating through a transition state (‡). Typical energies and distances are indicated. When the activation free energy for binding (ΔGa‡) is small, the system may cross the transition state multiple times (rapid rebinding) before irreversible escape to large radial separation occurs. (b) Three-state kinetic model for dissociation in the presence of rapid rebinding. On exit from the bound stateA·B,Bis initially in a region of space (orange shading) from which rapid rebinding toAcan occur. Irreversible escape occurs whenBleaves this region. (c) Three-state model in the presence of a competitor moleculeC(black).Cbinding toAprovides an additional reaction pathway that reduces the probability ofBrebinding toA. Figure 1a illustrates how the free-energy changes with radial separation for an example biological non-covalent interaction. We assume physiological ionic conditions under which electrostatic interactions are effectively screened for separations >~1 nm. The energy landscape has two roughly defined regions. When the radial separation is of the length scale set by non-covalent bonding interactions (on the order of a nanometre) or less, the shape of the landscape is determined by the details of the bonding interactions between the two binding partners. In contrast, at larger radial separations, the shape is independent of molecular details; the free energy falls off with radial separation simply because of the increased translational entropy of the separated partners in solution, which is proportional to the logarithm of the volume available to one partner at a particular radial separation from the other. Figure 1: Rapid rebinding of a bimolecular complex before full dissociation. ( a ) Schematic energy diagram for two binding partner molecules arbitrarily designated A (red) and B (green) dissociating through a transition state (‡). Typical energies and distances are indicated. When the activation free energy for binding (Δ G a ‡ ) is small, the system may cross the transition state multiple times (rapid rebinding) before irreversible escape to large radial separation occurs. ( b ) Three-state kinetic model for dissociation in the presence of rapid rebinding. On exit from the bound state A·B , B is initially in a region of space (orange shading) from which rapid rebinding to A can occur. Irreversible escape occurs when B leaves this region. ( c ) Three-state model in the presence of a competitor molecule C (black). C binding to A provides an additional reaction pathway that reduces the probability of B rebinding to A . Full size image The rates of biochemical dissociation and association reactions span many orders of magnitude [20] . The fastest association reactions approach the Smoluchowski limit [21] in which the second-order binding rate constant is determined only by the rate at which the two binding partners collide by diffusion through solution. Such fast rates imply that the free-energy barrier for association (Δ G a ‡ ) is small (on the order of the thermal energy k B T ). In such cases, the reaction trajectory can be complex. Even when one of the molecules has diffused a few nanometres away from its binding partner, beyond the reach of non-covalent bonding interactions (right side of Fig. 1a ), there is still a substantial probability it will be recaptured rather than escaping from its binding partner by diffusing away to long distances [4] . This probability gradually decreases as the radial separation increases. In general, the partners could rebind multiple times before they reach a radial separation large enough that they can be experimentally detected as unbound [15] , [16] . Calculations based on molecular diffusion have shown that the essential features of the reaction trajectory on a low activation barrier free-energy landscape similar to the one in Fig. 1a can be recapitulated with a simplified three-state model ( Fig. 1b ) [4] , [16] . To account for the effect of rapid rebinding, this model includes an ‘effective’ state ( A~B ) intermediate between the fully bound complex ( A·B ) and the unbound, freely diffusing partners ( A+B ). In this model, the system is considered to be in the A~B state when partner separation is greater than in the transition state (‡ in Fig. 1a ) but less than a characteristic length, σ ; σ is chosen to be the size of the region from which the probability of rebinding is substantial. The A~B state encompasses molecular configurations in which the partners have no energetically significant interactions with each other but are simply physically close. The three-state model ( Fig. 1b ) makes the prediction that the overall rate of dissociation (that is, the rate of production of A+B when starting from A·B ) is Where is the probability of recapture from the A~B state (refs 15 , 16 ). These predictions are predicated on the assumption that k a >> k d , which will be true for most biologically significant reactions with stable A·B complexes (that is, where Δ G a ‡ ≪ Δ G d ‡ , in Fig. 1a ). Given that B can rapidly rebind to its partner A , the addition of a competitor for binding to A would be expected to interfere with some rapid rebinding events and thereby increase the overall rate of dissociation. In the simple three-state model, the competitor effect can be included by postulating that competitor binding competes for rapid rebinding of B to A and adds an additional path for dissociation, as shown in Fig. 1c . The additional dissociation path reduces in a competitor concentration-dependent manner the rebinding probability: . Here, k on is the second-order rate constant for competitor binding and c is the competitor concentration. Substituting p r ( c ) into equation (1) leads to the prediction that the rate of dissociation increases with competitor concentration: In the limit of very large c (that is, k on c >> k esc + k a ) the dissociation rate tends to k d , while at low c the rate increases linearly with competitor concentration. In addition to the three-state model, which approximates the effect of rapid rebinding using the A~B effective state, we also considered a model that explicitly takes into account diffusion of the three molecular species (see ‘Diffusion model of rapid rebinding’ in Methods). We found that the diffusion model predicts an effect of competitor on the rate of dissociation that is quantitatively similar to the three-state model, but has a different functional form (see ‘Comparison of diffusion and three-state models’ in Methods). The key conclusion from either model is that the rate constant of bimolecular complex dissociation k off increases with increasing competitor concentration because of competitor interference with rapid rebinding. Single molecule imaging of competitor-induced dissociation The above theory predicts that competitor-accelerated dissociation is a general phenomenon that should apply to all bimolecular complexes. To test the theory, we studied as a specific model system the dissociation of duplex DNA. This system was chosen because it is a well-understood reaction in which one can rule out alternative mechanisms for competitor-accelerated dissociation kinetics. In particular, the formation of specifically base-paired ternary complexes can be avoided by choice of experimental conditions [22] , [23] , [24] . In addition, the formation of kinetically significant non-base-paired encounter complexes is unlikely due to electrostatic repulsion. We studied the dissociation reaction using a multi-wavelength co-localization single molecule technique in which the dissociation can be directly observed [25] , [26] . The experiments can accurately measure dissociation kinetics both in the absence of competitor and at varying concentrations of competitor. Moreover, the single molecule dissociation measurements are spatially resolved. At the low DNA surface density used in the experiments, they can distinguish rebinding to the same surface-tethered molecule from rebinding to a different molecule, the mechanism previously established for cell receptors at high surface density. To test the prediction that the apparent first-order dissociation rate constant k off ( c ) of a bimolecular complex increases with competitor concentration c , we used the experimental design shown in Fig. 2a . We tethered to the surface of a microscope flow chamber binding partner A , a 42-bp duplex DNA tagged with a red fluorescent dye, which has a 12-nt single-stranded extension ( Supplementary Fig. 1 ). Next, we formed bimolecular complexes between these molecules and molecules of binding partner B , a green dye-tagged, 8-nt single-stranded DNA ( Supplementary Fig. 1 ) complementary to the central 8 nt of the 12-nt single-stranded region of A . After complex formation, remaining unbound B was washed from the chamber. Using total internal reflection fluorescence microscopy, we observed the A·B complexes, which appeared as co-localized spots of red and green fluorescence ( Fig. 2b ). Spontaneous dissociation of an individual complex was detected as the disappearance of the green ( B ) fluorescence spot ( Fig. 2b and Supplementary Movie 1 ). We recorded the fraction of bound B molecules remaining at different times after the wash step. The resulting survival curve was exponential and a fit to the data (see Methods) yielded the dissociation rate constant k off in the absence of competitor ( Fig. 2c ). The average value of this rate constant was 0.017±0.001 s −1 (s.d., N =4 replicates). 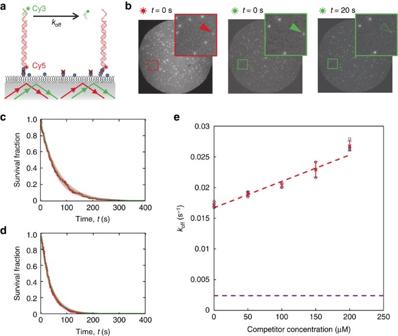Figure 2: Rate of dissociation of a DNA duplex measured in a single-molecule experiment. (a) Experimental design. Binding partnerA(red), a double-stranded DNA with a single-stranded extension labelled with the red dye Cy5, was tethered to a PEG-derivatized surface by a biotin/streptavidin/biotin linkage (blue/brown/blue). Dissociation fromAof binding partnerB(green), a single-stranded oligonucleotide labelled with the green dye Cy3, occurred spontaneously with rate constantkoff. The sample was imaged using total internal reflection fluorescence excitation with red and green lasers (arrows). (b) Images of the same microscope field of view (60 μm × 60 μm) ofA(red dye) andB(green dye) taken at the beginning of the experiment or 20 s after, as indicated. Insets show magnified views of the marked regions. Filled arrowheads denoteAandBfluorescent spots that were co-localized att=0; att=20 s, theBspot was absent (open arrowhead). (c) Fraction of theBspots that co-localized withAat the beginning of the experiment and survived at various times after the beginning of the experiment (red line; shaded region is 95% confidence interval (CI)). An exponential survival curve (green) withkoff=0.017 s−1(95% CI: [0.015, 0.019]) determined by fitting theBspot lifetimes (see Methods) is shown. (d) Same as incbut for an experiment in which 200 μM unlabelled competitor with the same nucleotide sequence asBwas added.koff=0.027 s−1(95% CI: [0.025, 0.032]). (e) Measuredkoffvalues (○) in replicate experiments (N=2–4) and their mean±s.e.m. ( × ) at various competitor concentrations. Line is a weighted linear fit with slope 4.31 × 10−5μM−1s−1. The calculated upper limit of the photobleaching rate is indicated (dashed magenta line). Figure 2: Rate of dissociation of a DNA duplex measured in a single-molecule experiment. ( a ) Experimental design. Binding partner A (red), a double-stranded DNA with a single-stranded extension labelled with the red dye Cy5, was tethered to a PEG-derivatized surface by a biotin/streptavidin/biotin linkage (blue/brown/blue). Dissociation from A of binding partner B (green), a single-stranded oligonucleotide labelled with the green dye Cy3, occurred spontaneously with rate constant k off . The sample was imaged using total internal reflection fluorescence excitation with red and green lasers (arrows). ( b ) Images of the same microscope field of view (60 μm × 60 μm) of A (red dye) and B (green dye) taken at the beginning of the experiment or 20 s after, as indicated. Insets show magnified views of the marked regions. Filled arrowheads denote A and B fluorescent spots that were co-localized at t =0; at t =20 s, the B spot was absent (open arrowhead). ( c ) Fraction of the B spots that co-localized with A at the beginning of the experiment and survived at various times after the beginning of the experiment (red line; shaded region is 95% confidence interval (CI)). An exponential survival curve (green) with k off =0.017 s −1 (95% CI: [0.015, 0.019]) determined by fitting the B spot lifetimes (see Methods) is shown. ( d ) Same as in c but for an experiment in which 200 μM unlabelled competitor with the same nucleotide sequence as B was added. k off =0.027 s −1 (95% CI: [0.025, 0.032]). ( e ) Measured k off values ( ○ ) in replicate experiments ( N =2–4) and their mean±s.e.m. ( × ) at various competitor concentrations. Line is a weighted linear fit with slope 4.31 × 10 −5 μM −1 s −1 . The calculated upper limit of the photobleaching rate is indicated (dashed magenta line). Full size image As the concentration of free B in the bulk solution is negligible in this experiment (see Methods), and also as we only analyse A·B complexes that are present at the onset of the experiment, reduction of the apparent dissociation rate by binding of B from bulk solution to A is excluded. In addition, a separate experiment ( Supplementary Fig. 2 ) showed no detectable photobleaching (the measured rate of photobleaching was 0.0002, s −1 , with an upper bound of the 90% confidence interval equal to 0.0024, s −1 ); thus, photobleaching makes at most only a negligible (<~15%) contribution to the measured rate constant. To measure the effect of competitor on the dissociation rate constant, we repeated the same experiment with the addition of various (up to 200 μM) solution concentrations of a competitor oligonucleotide ( Supplementary Fig. 1 ) identical to B , except that it lacked the dye label. The presence of competitor clearly increased the A·B dissociation rate k off (for example, Fig. 2d ). The dependence of the measured dissociation rate on competitor concentration is consistent with the three-state ( Fig. 2e ) and the diffusion ( Supplementary Fig. 3 ) models in the limit when the number of rebinding events is large (see Discussion). No significant dissociation through a ternary intermediate The mechanisms that we have discussed so far do not take into account the possibility that the two binding partners and the competitor can form a ternary complex A·B·C that contains all three molecules simultaneously. The formation of a ternary complex provides an alternative ‘displacement’ pathway for binding partner dissociation that can cause a competitor concentration dependence of k off , which is independent of the competitor inhibition of rapid rebinding predicted by the above theory. It is noteworthy that the A·B·C complex is a real state, corresponding to a minimum in the free-energy landscape. This real state is distinct from the A~B effective state ( Fig. 1b ), which does not contain competitor and merely represents freely diffusing A and B molecules that have a substantial probability of rebinding. We chose duplex DNA dissociation as the system with which to test the theory because the structure of the ternary complex in competitor-induced DNA strand release is known and the maximum extent to which it contributes to the dissociation rate is quantitatively understood [22] , [23] , [24] . In particular, the ternary complex intermediate for strand release in our experiment would arise when base pairs at one end of the A·B duplex spontaneously break, leaving a single-stranded DNA portion of A free to hybridize with one end of an incoming competitor molecule ( Fig. 3a ). The resulting three-stranded complex would then subsequently resolve in a random walk ‘zippering’ motion in which either the competitor fully replaces the B strand, releasing free B into solution, or the competitor is displaced by B , regenerating the starting A·B duplex ( Supplementary Fig. 4a , bottom). 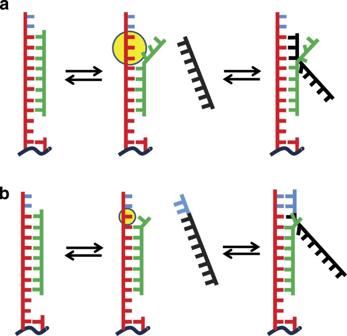Figure 3: Toehold experiment. The figure illustrates the design of a toehold experiment to exclude strand displacement through a ternary complex. (a) If competitor-induced strand displacement were to occur through a ternary complex, the rate-limiting step would be the melting (highlighted yellow) of three base pairs between theA(red) andB(green) DNA strands22. Melting could occur at either end of the duplex. CompetitorC(black) would then base pair withA, forming a ternary complex (right). Note thatBandChave identical sequences and thatCcannot base pair with the two-nucleotide single-stranded segments flanking theA·Bduplex (seeSupplementary Fig. 1). (b) The 10-nt competitorEC5(black/blue) can form additional base pairs with a two-nucleotide single-stranded DNA (blue) toehold adjacent to theA·Bduplex. Consequently, ifEC5could act through a strand-displacement mechanism, the rate-limiting step to form a ternary complex strand displacement intermediate is melting of only a single base pair (highlighted yellow). The same is true forEC3(not shown), which uses a 2-nt toehold at the opposite end of theA·Bduplex. Figure 3: Toehold experiment. The figure illustrates the design of a toehold experiment to exclude strand displacement through a ternary complex. ( a ) If competitor-induced strand displacement were to occur through a ternary complex, the rate-limiting step would be the melting (highlighted yellow) of three base pairs between the A (red) and B (green) DNA strands [22] . Melting could occur at either end of the duplex. Competitor C (black) would then base pair with A , forming a ternary complex (right). Note that B and C have identical sequences and that C cannot base pair with the two-nucleotide single-stranded segments flanking the A·B duplex (see Supplementary Fig. 1 ). ( b ) The 10-nt competitor EC5 (black/blue) can form additional base pairs with a two-nucleotide single-stranded DNA (blue) toehold adjacent to the A·B duplex. Consequently, if EC5 could act through a strand-displacement mechanism, the rate-limiting step to form a ternary complex strand displacement intermediate is melting of only a single base pair (highlighted yellow). The same is true for EC3 (not shown), which uses a 2-nt toehold at the opposite end of the A·B duplex. Full size image In our dissociation rate measurements ( Fig. 2 ), we chose the length of the A·B duplex, the competitor concentration range and the reaction temperature to make the fraction of the molecules that dissociated through the displacement pathway negligible. The data of Reynaldo et al. [22] yield an estimate ( Supplementary Fig. 4b,c ) that adding competitor under the conditions we used will cause at most a small minority of the molecules to dissociate using the displacement pathway, resulting in a 7.5% increase in the dissociation rate when competitor concentration is increased from 0 to 200 μM. The 57±2% increase we observe ( Fig. 2e ) as we increase the competitor concentration from 0 to 200 μM is much larger, indicating that it cannot be explained by the displacement mechanism. This is consistent with our proposal that the competitor-induced increase in k off that we observe is caused by inhibition of rapid rebinding, a mechanism which is independent of ternary complex formation. Note that the estimate of a 7.5% increase in the dissociation rate to 200 μM competitor assumes that the competitor concentration dependence observed by Reynaldo et al. [22] is solely due to the displacement pathway (as is illustrated in Supplementary Fig. 4a ). To the extent that inhibition of rapid rebinding results in a competitor dependence of the spontaneous dissociation pathway (as we propose here), the data of ref. 22 would yield a yet lower estimated contribution of the displacement pathway. To supplement the above argument, we sought an independent experimental test to confirm that formation of an A·B·C ternary complex does not explain the competitor dependence of the measured k off values in our experiments. Three-colour co-localization experiments are unlikely to directly observe A·B·C , because it is too short lived [27] , and also because the solution C concentrations needed ( Fig. 2e ) are too high to permit single-molecule detection of the complex [28] . Instead, we performed toehold exchange experiments [23] , [24] in which we examined k off in the presence of a competitor that is complementary to the single-stranded portion of A , but is two nucleotides longer than C ( Fig. 3b ). With the original competitor lacking the toehold, the rate-limiting step for the displacement pathway is the melting of 3 bp of the A·B duplex followed by formation of a 3-bp A·C duplex [22] , [29] , [30] ( Fig. 3a ). The rate-limiting step for the displacement pathway with the extended competitor requires melting of only one A·B base pair ( Fig. 3b ) and is therefore expected to be 12-fold faster (see Methods). In separate experiments with 200 μM of competitors that have the two-nucleotide extension on either the 5′ ( EC5 in Supplementary Fig. 1 ) or 3′ ( EC3 in Supplementary Fig. 1 ) end, we measured k off =0.026±0.003 s −1 and 0.036±0.005 s −1 , respectively, clearly not the 12-fold increase expected from the displacement pathway. Indeed, the dissociation rate measured in the presence of 200 μM EC5 is indistinguishable within the limits of experimental uncertainty to that measured with 200 μM C ( k off =0.027±0.001 s −1 , Fig. 2d ), whereas 200 μM EC3 shows a small but possibly significant increase over 200 μM C . These data suggest that with the non-extended competitor C , the ternary complex pathway accounts for at most 5% of the total dissociation at 200 μM C (see Methods). This small value is roughly consistent with 7.5% estimate from literature data [22] discussed above. This negligible amount of dissociation by the displacement pathway cannot account for the 57±2% increase in rate when c is increased from 0 to 200 μM ( Fig. 2e ). Thus, this second line of evidence again shows that the displacement mechanism does not cause the competitor concentration dependence of the dissociation rate that we observe in Fig. 2e . In this study, we consider a simplified three-state kinetic model and an explicit diffusion model for the dissociation of a bimolecular complex in the presence of competitor. The two models use different approaches to account for competitor interfering with the rapid rebinding that slows the overall rate of complex dissociation. Both models produce quantitatively similar predictions that the dissociation rate of a bimolecular complex will increase with increasing concentration of competitor. This is a general conclusion that does not depend on the molecular details of the interactions between the two binding partners. The prediction is confirmed by our experiments on a model bimolecular complex consisting of base-paired DNA strands. The competitor effect is significant even at biologically relevant (sub-millimolar) concentrations and control experiments confirm that the observed effect is independent of ternary complex formation. The simple conclusion from the experiments is that the rate of dissociation increases linearly with competitor concentration. Does this agree with the three-state model? As long as there are many rebinding events preceding a dissociation event, the model ( Fig. 1b ) predicts that the average number of rebinding events is related to the probability of rebinding (see ref. 15 ). Therefore, the limit of many rebinding events (‹ N ›>>1) corresponds to the probability of rebinding ( p r ) being close to 1. In this limit, the dissociation rate is strongly affected by rebinding (equation 1) and is given by k off ≈ k d /‹ N ›. Furthermore, in the presence of competitor ( Fig. 1c ), this limit corresponds to k a >> k esc + k on c , and equation (2) simplifies to Thus, if there are many rebinding events preceding a dissociation, the three-state model predicts a linear dependence of the dissociation rate with competitor concentration ( c ) in agreement with the experimental observations ( Fig. 2e ). The diffusion model predicts a different functional form but one that is also consistent with our observations (see ‘Comparison of diffusion model to experimental data’ in Methods). The model and the experimental measurements together yield an estimate of the rapid rebinding region size. The three-state model posits an A~B ‘effective state’ ( Fig. 1b,c ) encompassing molecular configurations in which the two binding partners have no energetically significant interaction but are close enough that the probability of B rebinding to the immobilized A (instead of diffusing away) is substantial. The radius σ of the rapid rebinding region figures in two of the rate constants in the three-state model ( Fig. 1b,c ). First, the rate constant for escape of the B from this region is set by the typical time to diffuse a distance σ , and is thus approximately k esc ~ D / σ 2 where D is the diffusion constant of B . Second, in the many rebinding limit k a >> k esc + k on c described above, the competitor binding rate is limited by the rate at which competitor in bulk solution enters the rapid rebinding region. This rate is approximated by the Smoluchowski formula k on =4 πDσ , assuming the competitor has the same diffusion constant as B (as is the case in our experiments). By taking the ratio of k on and k esc , the diffusion constant drops out and we arrive at the relationship In the case of many rebinding events, theory predicts a linear dependence of k off on c such that the ratio of the slope to intercept is equal to k on /k esc (equation 3). We observe the linear relationship in our experiments ( Fig. 2e ) and find slope/intercept ≈2,600 M −1 , allowing us to use equation (4) to estimate σ ≈7 nm. This is only an approximate estimate, as the assumptions of the Smoluchowski treatment (for example, spherical molecules with fully reactive surfaces) are not fully valid for the molecules used in the experiments. Nevertheless, the result that σ is on the order of the physical size of the molecules A and B is consistent with the prediction of a simple diffusion-to-capture calculation, which shows that the capture probability approaches one as the distance to the absorber centre approaches the absorber radius [31] . At 200 μM, the highest concentration of competitor used in the experiments, the rebinding region, a sphere of radius σ =7 nm will on average contain on the order of one competitor molecule. It makes sense that at this concentration competitor can interfere with rapid rebinding of B . Thus, based on two independent estimates, we conclude the value of σ extracted from the experimental data is consistent with the proposed mechanism of acceleration of bimolecular complex dissociation by occlusion of rapid rebinding. Taken together, the theory and experimental results are consistent with the rapid rebinding model of bimolecular dissociation. In the absence of competitor, the functional form of the dissociation kinetics is that predicted by a simple two-state (bound and free) kinetic mechanism, consistent with previous Brownian dynamics calculations [15] . Adding sufficiently high competitor concentrations unmasks the effects of rapid rebinding. The competitor interferes with rapid rebinding in a concentration-dependent manner, leading to a concentration-dependent dissociation rate constant k off . In many studies of the dissociation of a bimolecular complex, the observation of concentration-dependent dissociation rates has been taken as evidence, sometimes as the only evidence, for the existence of a ternary complex between the binding partners and competitor that could not be directly observed. Our work raises the possibility that the competitor dependence in some of these systems is not due to ternary complex formation. Instead, the competitor dependence may arise from competitor interference with rapid rebinding. Our work sets the concentration scale over which this effect can become significant and thus provides a quantitative framework for distinguishing reactions that use ternary complex-mediated versus simple dissociation molecular mechanisms. In particular, inhibition of rapid rebinding can become significant when competitor concentration is high enough that the mean distance between competitor molecules is on the order of the size of the binding partners. To calculate the size of the competitor effect requires detailed knowledge of the molecular shapes, binding geometries and the shape of the energy landscape at the molecular scale. Competitor concentration dependence of dissociation rates has been previously reported for complexes between proteins and DNA. For proteins that bind to DNA in a sequence nonspecific fashion, Graham et al. [7] proposed that the concentration dependence may be explained by ‘micro-dissociation’ of the protein–DNA complex, where the micro-dissociated (positively charged) protein remains near the (negatively charged) DNA due to long-range electrostatic forces. Such weakly bound electrostatic complexes or other postulated ‘encounter complexes’ (see ref. 32 and literature cited therein) are unlikely to play a role in our experiments, where both binding partners and the competitor are negatively charged. In a subsequent study, Sidorova et al. [9] examined a protein capable of both sequence-specific and nonspecific interactions with DNA. They concluded that the ionic strength dependence excluded a ternary complex mechanism for the competitor concentration dependence of the dissociation rates, and favoured a model based on competitor interference with nonspecific rebinding. In both of these studies, the presence of a large number of nonspecific sites on the same DNA molecule may have caused competitor interference with rapid rebinding to occur in a competitor concentration range that is lower than that seen in our experiments, in which only a single specific binding site was present (see Methods). A similar phenomenon explains some competitor-accelerated dissociation of ligands from cell membranes that contain large numbers of receptors (see the introduction). The studies presented here have significant implications for measurements of dissociation rates in single-molecule co-localization experiments. Single-molecule fluorescence co-localization experiments have been used as an alternative to bulk measurements in quantitatively characterizing dissociation kinetics in a variety of protein and nucleic acid systems (for example, refs 25 , 26 , 33 , 34 , 35 , 36 , 37 ). Such experiments detect dissociation on time and distance scales which are limited by the temporal and spatial resolution of the microscope. When used to study single fluorescent molecules, the spatial resolution can approach 1 nm, but the time resolution is typically restricted to a millisecond or poorer. These resolution limits are larger and slower, respectively, than those typical for breakage of non-covalent bonds between molecules. Therefore, the dissociation rate constants measured in these experiments might depend on the microscope resolution and in principle differ from those measured in bulk competition experiments. Thus, correct interpretation of such single-molecule dissociation measurements requires explicit consideration of the diffusion of the molecular components. Based on the size of the rapid rebinding region estimated from our experiments ( σ =7 nm) and the diffusion constant D =150 μm 2 s −1 (refs 38 , 39 , 40 ), we can also estimate the characteristic time for escape of the B strand from this region as 1/ k esc =0.3 μs. This is orders of magnitude faster than the time resolution of typical single-molecule co-localization experiments. As 1/ k esc places an upper bound on the lifetime of the effective A~B state, co-localization experiments are incapable of directly detecting the rapid rebinding of A and B after they dissociate. Instead, they detect the effective dissociation rate that includes the effects of undetected rapid rebinding. Thus, the theory and experimental results reported here confirm that the dissociation rates measured in the single-molecule experiments either with or without competitor are expected to be identical to those measured in conventional bulk dissociation measurements. What is the role of rapid rebinding in living cells? A noteworthy result from these studies is that the phenomenon of acceleration of dissociation by interference with rapid rebinding occurs at molecular concentrations that are relevant to pharmacology and cell biology. Slow dissociation of non-covalently bound complexes can be a key determinant of biological function [41] . In living cells, many proteins are present at low (nanomolar or sub-nanomolar) concentrations. On the other hand, to form stable, well-populated associations with their partners, proteins must bind with high equilibrium affinity. However, this implies slow dissociation, which may be incompatible with rapid biological responses. One solution to these competing requirements is to have binding competitors that can act to accelerate the dissociation of high-affinity interactions [7] . There are well-studied examples in which such dissociation is accelerated by formation of a ternary complex between the protein, its binding partner and the competitor [10] , [11] , [12] , [42] . However, our work demonstrates that formation of a ternary complex is not necessary to have competitor-accelerated dissociation. Here we show that even sub-millimolar concentrations of competitor are sufficient to significantly accelerate dissociation of a macromolecular complex without ternary complex formation. Microscopy Single-molecule fluorescence microscopy was performed on a micro-mirror multi-wavelength total internal reflection fluorescence microscope described previously [25] , [36] . Sample temperature was maintained at 28±0.5 °C using a custom temperature-control system that heated the stage and the objective mount. Images (1 s duration frames collected every 2 s) were recorded with simultaneous excitation of 150 μW at 532 nm and 75 μW at 633 nm (excitation powers measured incident to the objective back aperture). Lasers were shuttered except during image acquisition. Sample preparation DNA oligonucleotides with the structures shown in Supplementary Fig. 1 were obtained from Integrated DNA Technology. Flow chambers (typical volume 20–25 μl) were constructed as previously described [25] , with the following modifications: glass cover slips (Gold Seal 24 × 60 mm No. 1.5 and 25 × 25 mm No.1) were used instead of fused silica cover slips, and the derivatization procedure used a 200:1 ratio of PEG-SVA5000 to biotin-PEG-SVA5000 (both from Laysan Bio). The polyethylene glycol (PEG) derivatization of the cover slips serves to minimize interactions of the DNA with the surface [43] . The chamber was first washed with 2 × 120 μl microscopy buffer (MB) consisting of 75 mM NaCl, 40 mM Tris–Cl, 0.2 mM EDTA, 0.1% w/v albumin, BSA (EMD Chemicals) adjusted to pH 8.0. Next, the chamber was incubated for ~40 s in 0.013 mg ml −1 streptavidin (Invitrogen) in MB. After removing the free streptavidin with 2 × 120 μl MB, biotinylated A DNA at 20 pM in MB supplemented with an oxygen scavenging system (OS; 10 mM dithiothreitol, 15 mM glucose, 0.02 mg ml −1 catalase, 0.1 mg ml −1 glucose oxidase [36] ) was introduced and incubated for a total of ~10 s; the desired surface density of labelled A (200–250 molecules per ~60 μm diameter field of view) was confirmed by brief (~2 s) imaging. The incubation was terminated by washing with 2 × 120 μl MB+OS. Next, the chamber was incubated with 2.5 nM B DNA in MB+OS supplemented with 2.3% (w/v) PEG 8000 for 1–2 min to form A·B complexes. The dissociation reaction was initiated by washing over ~10 s with 120 μl MB+OS+PEG, either alone or supplemented with the specified concentration of unlabelled competitor DNA. Termination of the wash step was taken to be time t =0 for the reaction. Data analysis Images from the total internal reflection fluorescence microscope were obtained and processed with custom LABVIEW and MATLAB software. The surface positions of each green spot ( B molecule) that co-localized with a red spot ( A molecule) were recorded at time zero. The lifetime of each of these green spots was determined by examining successive images ( Fig. 4 ). During the dissociation experiment, B was present in the solution at a low residual concentration. However, this residual B bound to unoccupied A at a rate of only 1.5 × 10 −4 s −1 (19 events detected on 322 DNA molecules over 400 s) which is negligible compared with the measured dissociation rates. This, together with the fact that only spots present at time zero were scored, ensures B binding from bulk solution does not alter the measured dissociation rate constants. Typically, ~98% of spots disappeared during the observation time (200–400 s); spots that remained were excluded from subsequent analysis. The collected spot lifetimes from a recording were fit assuming an exponential survival fraction f ( t )=exp(− k off t ) using a maximum likelihood algorithm, yielding the dissociation rate constant k off . Confidence intervals for the rate constants and the theoretical survival function were determined by bootstrapping. The s.d. of rate constants measured in replicate experiments conducted on different days (for example, error bars in Fig. 2e ) were similar in size to the s.e. in the individual measurements estimated from the bootstrap analysis, indicating that there were no systematic differences between replicates larger than the statistical uncertainty in the individual measurements. For example, for the five replicate measurements of the dissociation rate constant at zero competitor concentration ( Fig. 2e ), the s.d. of the measurements was 0.001 s −1 , while the s.e. of the individual measurements (for example, that shown in Fig. 2c ) was 0.002 s −1 . All uncertainties reported in the text are s.d. calculated from three to four replicated measurements unless otherwise specified. 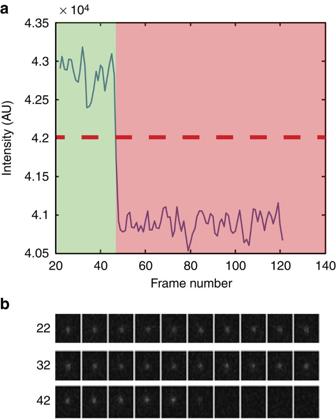Figure 4: Scoring dissociation in a total internal reflection fluorescence experiment. Example fluorescence intensity record (a) and corresponding images (b; frames 22 through 51) showing disappearance of a single Cy3-labelledBmolecule bound to a surface-tetheredAmolecule. The record starts after washing the flow chamber with buffer (frame 22), which is taken to bet=0. Preliminary detection of spot disappearance used crossing of an intensity threshold (red broken line) chosen to be well separated from the signal and background intensities for a particular recording. However, in all cases we checked that the events corresponded to disappearance of a discrete spot of fluorescence well centred on the DNA position (at frame 47 in the example shown). Figure 4: Scoring dissociation in a total internal reflection fluorescence experiment. Example fluorescence intensity record ( a ) and corresponding images ( b ; frames 22 through 51) showing disappearance of a single Cy3-labelled B molecule bound to a surface-tethered A molecule. The record starts after washing the flow chamber with buffer (frame 22), which is taken to be t =0. Preliminary detection of spot disappearance used crossing of an intensity threshold (red broken line) chosen to be well separated from the signal and background intensities for a particular recording. However, in all cases we checked that the events corresponded to disappearance of a discrete spot of fluorescence well centred on the DNA position (at frame 47 in the example shown). Full size image Contribution of the displacement pathway to dissociation The rate-limiting step for DNA duplex dissociation through the displacement pathway ( Supplementary Fig. 4a , bottom) is the melting of 3 bp and subsequent binding of competitor leading to the formation of a stable ternary complex A·B·C ( Fig. 3a ) [22] , [23] , [29] , [30] , [44] . To estimate the contribution of this pathway to the overall dissociation reaction, we designed extended competitors EC3 and EC5 ( Supplementary Fig. 1 ), which can form a stable 3-bp ternary complex when only a single bp of the original duplex has melted ( Fig. 3b ). Reynaldo et al. [22] showed that the rate constant for competitor association, the rate-limiting step of the displacement pathway, is where k c is the association rate constant for competitor binding to A , N is the length (in bp) of B , n is the number of base pairs needed to be melted to form a stable ternary complex (3 for C ; 1 for EC3 or EC5 ), Δ H is the enthalpy for melting those base pairs (taken from refs 45 , 46 ), T is the absolute temperature and R is the universal gas constant. T m =336 K, the melting temperature of a long duplex with the same G+C content as A·B , was calculated for the 75-mM NaCl conditions used in the experiments as described [47] . Assuming k c to be the same for C , EC3 and EC5 , equation (5) predicts that the displacement pathway should be 12-fold faster with extended competitors EC3 and EC5 than with competitor C under the experimental conditions used (28 °C and 75 mM NaCl). To estimate the contribution of the displacement pathway to the overall dissociation rate, we expressed the measured rate as k obs = k 0 + ck rr + ck 2 , where k 0 is the rate of spontaneous dissociation in the absence of competitor and ck rr is the additional rate of spontaneous dissociation caused by C interference with rapid rebinding, which is proportional to competitor concentration c (equation (3)). Similarly, the observed rate in the presence of EC3 or EC5 can be written as k′ obs = k′ 0 + ck′ rr + ck′ 2 , where we estimate k′ 2 =12 k 2 as described above. Simultaneous solution of these equations using the k obs values measured for zero competitor and 200 μM C , and the k′ obs value measured for 200 μM EC3 or EC5 yields estimates of the contribution of the displacement pathway to the overall dissociation rate at 200 μM C of 3.2±1.8% (using the EC3 data) and −0.3±1.1% (for EC5 ), indicating that the contribution is negligible. Diffusion model of rapid rebinding Rapid rebinding occurs when binding partners A and B dissociate but remain sufficiently close so that the probability of rebinding is large. The physics of rapid rebinding can be captured with a simple diffusion model in which A is an absorbing sphere of radius R (approximately equal to the sum of the radii of the two binding partners), and the B (binding partner) and C (competitor) molecules are point particles diffusing with a diffusion coefficient D (equal to the sum of the A and B diffusion coefficients); see Fig. 5 . Here we make the simplifying assumption, corresponding to the case in our experiments, that B and C have the same size and diffusion coefficient. 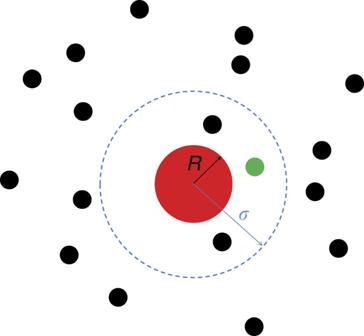Figure 5: Diffusion model of rapid rebinding. After disassociating from its binding partnerA(red sphere of radiusR), moleculeB(green) finds itself in the rapid rebinding region (dashed circle) of radiusσ. The space outsideAis also occupied by competitor moleculesC(black) initially at a uniform concentration. Both theBandCmolecules diffuse until one is captured byA. The probability thatBwill rebind before being excluded byCdecreases with increasingCconcentration, leading to a competitor-dependent dissociation rate. Figure 5: Diffusion model of rapid rebinding. After disassociating from its binding partner A (red sphere of radius R ), molecule B (green) finds itself in the rapid rebinding region (dashed circle) of radius σ . The space outside A is also occupied by competitor molecules C (black) initially at a uniform concentration. Both the B and C molecules diffuse until one is captured by A . The probability that B will rebind before being excluded by C decreases with increasing C concentration, leading to a competitor-dependent dissociation rate. Full size image When B dissociates from A (with rate constant k d ), we assume that it is initially in the rapid rebinding region, which we model as a sphere of radius σ > R . Initially, competitor molecules are assumed to be uniformly distributed in space at concentration c . Further, assuming that the effective overall dissociation rate constant ( k off ) is much less than the microscopic dissociation rate constant ( k d ), we showed above (equation 1) that the off rate is k off = k d [1− p r ( D , c , R , σ )]= k d p exit ( D , c , R , σ ), where p exit ( D , c , R , σ ) is the probability that B exits the rebinding region instead of rebinding to A . Next, we compute p exit ( D , c , R , σ ) in the diffusion model. The probability density that a diffusing particle ( B or C ) is at distance r ′ from the origin, assuming that there is an absorbing sphere of radius R at the origin and that the particle was at position r at time t =0 is (ref. 48 ): From this probability density, we can compute the probability of a particle being absorbed by the sphere at time t , which is equal to the probability flux into the absorbing sphere: If the particle is initially uniformly distributed in a spherical shell with radius R ≤ r ≤ σ , as we assume for B after it has disassociated from A , then the probability density of rebinding is obtained by averaging φ ( r , t ) over the spherical shell: For B to be able to rebind to A at time t , A must be free of competitor molecules. Therefore, the probability that B will rebind at any time after it has dissociated from A is where p u ( t ) is the probability that A has not captured a competitor molecule up to time t , that is, it is unoccupied by C at time t and free to bind B . To compute the survival probability p u ( t ) for A in a pool of competitors C at concentration c , we first compute the probability per unit time that a competitor binds to A at time t : The term in parenthesis can be interpreted as a time-dependent second-order rate constant [21] . At long times, it reduces to the well-known Smoluchowski steady-state rate constant k S =4 πDR . At short times, it is increased due to the presence of competitors that are by chance initially very close to A and are depleted in the steady state. In particular, the second term will dominate for , which is the characteristic time for a particle to diffuse over a distance comparable to the interaction radius. Assuming numbers that are typical of the reaction in our experiment, R =10 nm and D =100 μm 2 s −1 , this crossover time is . Using the probability density k ( t ), we can compute the survival probability of the unbound A as in ref. 21 : We now have both elements φ r ( t ) and p u ( t ) required in equation (9) to compute the probability p r that B will rebind after dissociating from A , and the probability of B exiting the rapid rebinding region p exit =1− p r . To better understand the competition between B and C that is encoded in equation (9), it is useful to introduce scaled, dimensionless variables , for the interaction radius, and , for the competitor concentration. If we also introduce dimensionless time , then substituting equations (8) and (11) into equation (9) yields We see that the result is independent of the diffusion constant. A three-dimensional plot of ( Fig. 6 ) is consistent with the physical picture of rapid rebinding and the effect of competitor that is provided by the three-state model we employed in the Results section. At large concentrations of competitor, p exit approaches 1. This is expected, as under those conditions C will bind A immediately after B has disassociated into the rapid rebinding region. At small competitor concentrations, p exit tends to a value that is determined by , the ratio of the interaction radius and the rebinding region size. When is close to 1, there will be multiple rebinding events and p exit approaches zero at low competitor concentrations. In this case, the apparent dissociation rate constant k off = k d p exit will be much smaller than the microscopic dissociation rate constant k d . Therefore, to observe a competitor-dependent dissociation rate constant we must be in the limit of many rebinding events, that is, σ ~ R . 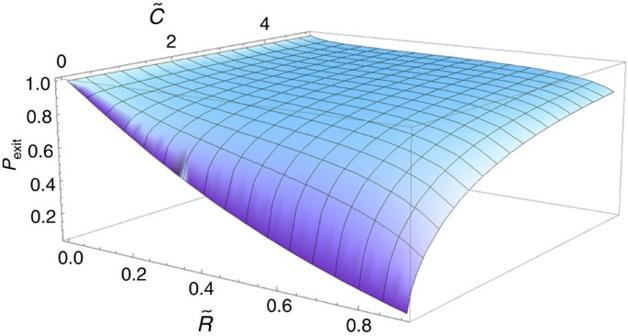Figure 6: Exit probability. The probability of exit from the rapid rebinding region for binding partnerBis plotted as a function of the scaled interaction radiusand the scaled competitor concentration. The exit probability approaches 1 at large-scaled concentrations. Significant variation in the exit probability, and therefore in the apparent dissociation constant, is only observed for scaled interaction radiusof order 1. Figure 6: Exit probability. The probability of exit from the rapid rebinding region for binding partner B is plotted as a function of the scaled interaction radius and the scaled competitor concentration. The exit probability approaches 1 at large-scaled concentrations . Significant variation in the exit probability, and therefore in the apparent dissociation constant, is only observed for scaled interaction radius of order 1. Full size image From Fig. 6 , we also conclude that to observe a competitor-dependent dissociation rate constant the concentration of competitor should be of the order of c ~1/ σ 3 (that is, ). For σ ~10 nm, as we believe to be the case in our experiments, c ~1 mM. In contrast, for the experiments in ref. 9 where a 360-bp DNA acts as antenna for binding a positively charged protein, σ ~100 nm, yielding σ ~1 μM as observed. Comparison of diffusion model to experimental data To determine whether the diffusion model predictions are consistent with our experimental observations, we fit the measured k off ( c ) values to k off = k d [1− p r ] where p r is given by equation (12). The fit corresponds closely to the data ( Supplementary Fig. 3 ). Estimation of the uncertainties in the parameter values by bootstrap analysis yielded bimodal parameter distributions. Presumably, this was due to inadequate constraints on the fit because the range of concentrations accessible in the experiments was not broad enough to include both the high and low regimes predicted when is close to 1 ( Fig. 6 ). The two subsets of bootstrap fits produced similar fit curves. In the first subset, R =3.3±0.1 nm, σ =3.3±0.1 nm and k d =68±23 s −1 . This corresponds to a non-physical situation in which the width of the rebinding region, ( R — σ ), is of sub-atomic dimensions, corresponding to a rebinding probability extremely close to 1. The other subset gave parameters R =3.8±0.3 nm, σ =4.0±0.7 nm and k d =0.8±0.3 s −1 . This result helps confirm that the model is a satisfactory explanation for the experimental data, as the R- and σ -values are of magnitudes that correspond to the physical size of the molecules studied. Furthermore, the value for σ is within a factor of 2 of that determined from the three-state model, despite the different character of that model and the assumptions on which it is based. Comparison of diffusion and three-state models The three-state model and the diffusion model both attempt to capture the physics of rapid rebinding without incorporating details of molecular interactions between the binding partners A and B . In the three-state model, this is achieved by introducing an effective A~B state in which molecule B is dissociated from molecule A but is in its close proximity and is therefore likely to rebind. The transitions into this state from the bound A·B state and out of it into the A+B state are assumed to occur at a constant probability per unit time, given by the rates k a and k esc , respectively. In this case, the probability of rebinding is . From this, the average number of rebinding events before dissociation into the A+B state is . In the diffusion model, we replace the effective A~B state with a spherical shell R < r < σ in which B finds itself after dissociating from A . The A molecule is modelled as a perfectly absorbing sphere of radius R , while σ is the radius of the rapid rebinding region. As in the three-state model, two parameters are introduced to characterize the physics of rapid rebinding. In the diffusion model, the number of rapid rebinding events can be computed using , the probability of rebinding for a diffusing particle placed at radius r > R to an absorbing sphere of radius R (ref. 49 ). Averaging this probability over all possible initial positions of B R < r < σ gives (as previously, ), from which the average number of rebinding events follows, as described above for the three-state model. Both models lead to the same conclusion that rapid rebinding reduces the dissociation rate from its microscopic value k d , which is the rate at which the bonds between A and B are broken, to an apparent dissociation rate . Both models are gross approximations of reality. On dissociating from A , its binding partner B will find itself at a distance from A on the order of a few nanometres. At that separation, the thermal motion of B will be affected by the complex interactions between B , its binding partner A and solvent molecules. The diffusion model ignores this and assumes no interactions, while the three-state model makes the assumption that the motion in the presence of these interactions leads to a simple constant in time rate of rebinding or escape. Still, the two models make quantitatively similar predictions as illustrated in Fig. 7 . 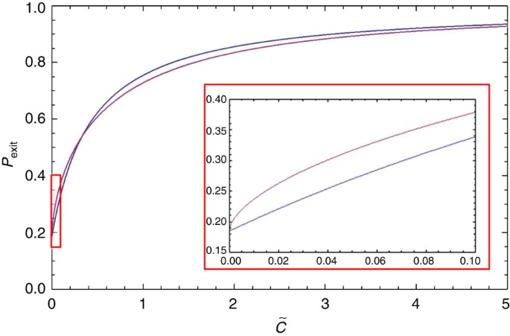Figure 7: Comparison of the three-state and diffusion models. The exit probability (pexit) calculated from the diffusion model (blue line) with the scaled interaction radius, for different values of the scaled competitor concentration. In violet, we show the calculation ofpexitbased on the three-state model with parameterska/kesc=4.41 and; the former was chosen so that both models have the same average number of rebinding events in the absence of competitor, while the latter is the estimated value from Results. The inset corresponds to the red rectangular area and shows the difference in the shapes of the two curves at low concentrations. Figure 7: Comparison of the three-state and diffusion models. The exit probability ( p exit ) calculated from the diffusion model (blue line) with the scaled interaction radius , for different values of the scaled competitor concentration . In violet, we show the calculation of p exit based on the three-state model with parameters k a / k esc =4.41 and ; the former was chosen so that both models have the same average number of rebinding events in the absence of competitor, while the latter is the estimated value from Results. The inset corresponds to the red rectangular area and shows the difference in the shapes of the two curves at low concentrations. Full size image Despite their quantitative similarity, the two models differ in the functional form of the dependence of the apparent dissociation rate constant on competitor concentration. This is visible at small concentrations, as illustrated in the inset of Fig. 7 where the diffusion model predicts an increase in k off that goes as the square root of the concentration, while the three-state model predicts a linear increase. For a physical bimolecular complex/competitor system, the precise functional form is likely to be different from that predicted by either model: it will depend on the details of the molecular geometries and of the interactions between the molecules on the nanometre scale. Still, the fact that two very different theoretical models of rapid rebinding give quantitatively similar predictions ( Fig. 7 ) and are both good at accounting for the experimental data (compare Fig. 2e and Supplementary Fig. 3 ) reinforces confidence in the universality of the competitor effect irrespective of details of the interactions between the binding partners. How to cite this article: Paramanathan, T. et al. A general mechanism for competitor-induced dissociation of molecular complexes. Nat. Commun. 5:5207 doi: 10.1038/ncomms6207 (2014).